Intestinal epithelial stem cells do not protect their genome by asymmetric chromosome segregation The idea that stem cells of adult tissues with high turnover are protected from DNA replication-induced mutations by maintaining the same 'immortal' template DNA strands together through successive divisions has been tested in several tissues. In the epithelium of the small intestine, the provided evidence was based on the assumption that stem cells are located above Paneth cells. The results of genetic lineage-tracing experiments point instead to crypt base columnar cells intercalated between Paneth cells as bona fide stem cells. Here we show that these cells segregate most, if not all, of their chromosomes randomly, both in the intact and in the regenerating epithelium. Therefore, the 'immortal' template DNA strand hypothesis does not apply to intestinal epithelial stem cells, which must rely on other strategies to avoid accumulating mutations. After semiconservative replication of eukaryotic chromosomes, each sister chromatid inherits one of the two original template DNA strands, and segregation of the new chromosomes between daughter cells is thought to occur randomly. However, past the period of rapid growth characteristic of development, the stem cells of some tissues are suspected to switch to a nonrandom mode of chromosome segregation (CS; reviewed in ref. 1 ). From that point of time onwards, one of the two template DNA strands of each chromosome, the 'immortal strand', according to the Cairns hypothesis [2] , is thought to be selectively and repeatedly transmitted to the 'stem' daughter cell, division after division ( Fig. 1a , asterisk), whereas the other template is inherited by the other, shorter-lived, daughter cell that will eventually migrate out of the stem compartment. This CS mode is assumed to prevent the accumulation of replication errors in the genome of stem cells [2] . Alternatively, if only a subset of chromosomes are involved, nonrandom CS could link the transmission of different epigenetic marks to differences in daughter-cell fate (reviewed in ref. 3 ). In several mammalian tissues, including the small intestine [4] , breast [5] , brain [6] and muscle [7] , [8] , nonrandom CS has been linked to self-renewing divisions of a fraction of stem cells. The main evidence provided in support of asymmetric CS in brain, breast and muscle cells was the observation of asymmetric label segregation in cultured cells. Two other experimental paradigms were examined in the intestine and the muscle: juvenile growth [4] , [7] and regeneration after injury in adult animals [4] , [7] , [8] . In the latter case, stem or progenitor cells of the injured tissue are assumed to transiently switch back to a symmetric mode of cell division involving random CS. This presumably enables incorporation of nucleic-acid base analogues into both DNA templates. Following the regenerative response, stem or progenitor cells are thought to resume nonrandom CS, and the repeated and selective inheritance of the 'immortal' strands is inferred from the long-term retention of labelled DNA in their nucleus, during successive divisions in the absence of label. 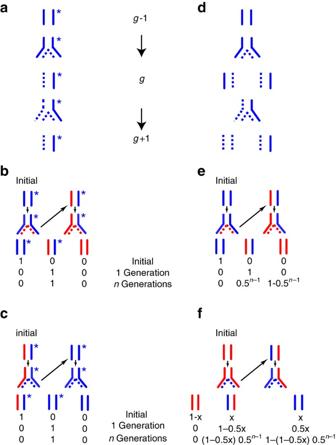Figure 1: Chromosome fates and labelling in the stem-cell lineages depending on the mode of chromosome segregation (CS). Solid lines represent parental template DNA strands and dotted lines represent newly synthesized strands. (a) Nonrandom chromosome segregation (CS) implies an asymmetric mode of cell division generating stem and non-stem daughter cells. The 'immortal' DNA template (*) inherited by a stem cell at generationg−1, is again inherited by the stem progeny at generationsgandg+1. (b) In the case of nonrandom CS, and no matter how long the labelling period (1 tongenerations), only one strand of each chromosome can be labelled (red) in stem cells as they systematically inherit the chromatid containing the initially unlabelled 'immortal' strand (blue*). (c) In the case of nonrandom CS, stem cells replicating their DNA in the absence of label are unlabelled from the first generation. (d) On the contrary, because random CS implies that both templates of generationg−1 can be transmitted to generationg+1 with equal probability, the proportion of labelled chromosomes steadily increases with each generation of stem cells produced in the presence of label (e), and steadily decreases with each generation of stem cells produced during the chase period (f). Figure 1: Chromosome fates and labelling in the stem-cell lineages depending on the mode of chromosome segregation (CS). Solid lines represent parental template DNA strands and dotted lines represent newly synthesized strands. ( a ) Nonrandom chromosome segregation (CS) implies an asymmetric mode of cell division generating stem and non-stem daughter cells. The 'immortal' DNA template (*) inherited by a stem cell at generation g −1, is again inherited by the stem progeny at generations g and g +1. ( b ) In the case of nonrandom CS, and no matter how long the labelling period (1 to n generations), only one strand of each chromosome can be labelled (red) in stem cells as they systematically inherit the chromatid containing the initially unlabelled 'immortal' strand (blue*). ( c ) In the case of nonrandom CS, stem cells replicating their DNA in the absence of label are unlabelled from the first generation. ( d ) On the contrary, because random CS implies that both templates of generation g −1 can be transmitted to generation g +1 with equal probability, the proportion of labelled chromosomes steadily increases with each generation of stem cells produced in the presence of label ( e ), and steadily decreases with each generation of stem cells produced during the chase period ( f ). Full size image The crypt of the intestinal epithelium is indeed seen as a potential candidate site for nonrandom CS because of its high cell turnover and capacity for regeneration sustained by a high number of stem cells [9] , [10] , as well as the fact that no quiescent intestinal stem cell has been identified so far, which could have a role of guardian of the genome [11] . However, the precise location of stem cells has long remained contentious (reviewed in ref. 12 ). Until very recently, the so-called cell position +4 (cp4) model placed stem cells at the base of the transit-amplifying progenitor compartment, just above the last Paneth cells in the small intestine [13] . The other model, supported by lineage studies [14] , [15] , assigned the status of stem cells to the immature proliferative crypt base columnar (CBC) cells intercalated between Paneth cells in the small intestine [16] . These cells were recently shown to express the leucine-rich repeat-containing G-protein-coupled receptor 5 (Lgr5) along the entire gastrointestinal tract [15] . Supporting both the cp4 model and the Cairns hypothesis was the finding that tritiated thymidine incorporated during post-irradiation crypt regeneration could be retained for at least 18 days in cycling cells, preferentially localized above Paneth cells [4] . Furthermore, some recently discovered multipotent stem cells expressing the B-cell-specific Maloney Murine Leukaemia Virus integration site 1 (Bmi-1) ring finger nuclear protein were reported to be preferentially located around cp4 (ref. 17 ). However, Bmi-1 is not expressed in the distal half of the small intestine and in the colon [17] , and its expression was later shown to overlap with that of several CBC stem-cell markers, including Lgr5 (refs 18 , 19 ). Hence, Bmi-1 and Lgr5 may mark overlapping cell populations. As CBC cells were shown to generate all epithelial lineages along the entire gastrointestinal tract, both in vivo [14] , [15] , [20] and in culture [21] , we decided to investigate their mode of CS in both the intact and regenerating intestinal epithelium of adult mice, and compare it with that of the neighbouring cp4 cells. Here we demonstrate that, unlike what is commonly thought, cp4 cells are not long-term label-retaining cells (LRCs) and our results suggest that both CBC and cp4 cells segregate their chromosomes randomly under homeostatic conditions and when recovering from a lesion. Defining the experimental approach The best available test capable of discriminating a nonrandom from a random CS mode involving all chromosomes is the DNA label dilution assay. The nonrandom CS mode has two implications, which are key to understanding the simulations described below. First, only one DNA strand per chromosome can be labelled in stem cells, regardless of the length of the labelling period ( Fig. 1a,b ). Second, all chromosomes of all stem cells should become unlabelled as soon as the 'immortal' strands serve as templates in the absence of label ( Fig. 1c , 1 generation). In contrast, both chromosome strands can be labelled in the case of random CS and the probability that all chromosomes become unlabelled after the first division occurring during the chase is negligible ( Fig. 1d–f ). Therefore, the fraction of labelled CBC cell nuclei detected after two or more cell cycles under both scenarios should mainly depend on two parameters, namely, the length of the labelling period relative to that of the cell cycle, and the threshold level of detection, hence explaining the importance of determining the cytokinetic parameters of CBC cells in order to optimize the labelling protocol and simulate the respective rates of decay in the labelling ratio under both scenarios. Cytokinetic parameters of CBC cells To determine the average duration of the CBC cell cycle, we subjected adult mice to a protocol of cumulative CldU labelling [22] . In an asynchronously distributed cell population, the proportion of CldU + cells scored after the first CldU pulse should reflect the length of the S phase ( Fig. 2a , solid black line) relative to the total length of the cell cycle (dotted cirle) [22] . Each new pulse of CldU labels cells that have entered the S phase since the last injection (red line). As a result, the fraction of labelled cells increases with time and a number (n) of pulses are needed to label all cycling cells. We then performed immunohistochemistry (IHC) on thin paraffin sections of rolled intestine, using Ki67 as a marker of cycling cells and phospho (ser10)-histone H3 to evaluate the percentage of cells in the G2/M transition. For cell scoring, we selected cells flanked by Paneth cells in longitudinal sections featuring part or all of the crypt lumen [23] . Analysis of the relationship between the ratio of CldU + Ki67 + CBC cells to the total number of Ki67 + CBC cells and time revealed a linear increase in labelled CBC cells until CldU labelling became saturated ( Fig. 2b ). It follows that CBC cells represent a single population in terms of S phase (9.4 h), G2/M phase (3.4 h) and cell cycle duration (28.5 h). 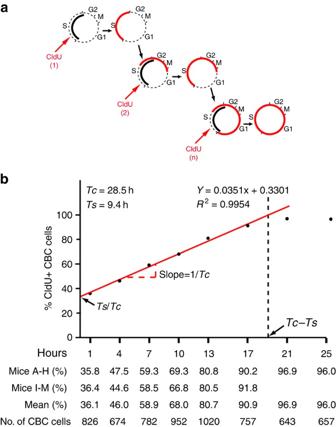Figure 2: Cytokinetic parameters of CBC cells. (a) Schematic representation of the protocol of cumulative CldU labelling. The solid black line represents the length of the S phase relative to the other phases of the cycle. The solid red line represents the distribution of cells within the cycle, which have been labelled with CldU. (b) Kinetics of cumulative CldU incorporation in CBC stem cells. We performed CldU immunohistochemistry on thin paraffin sections of rolled intestine, using Ki67 as a marker of cycling cells and phospho (ser10)-histone H3 to evaluate the percentage of cells in the G2/M transition. Analysis of the relationship between the ratio of CldU+Ki67+CBC cells to the total number of Ki67+CBC cells and time revealed a linear increase in labelled CBC cells until CldU labelling became saturated. Data points represent mean percentages of Ki67+CldU+CBC cell nuclei from two mice (A-F and I-M), except for the 21-h and 25-h time points (mice G,H). The average length of the cell cycle (Tc=28.5 h) is given by the slope of the regression line (1/0.0351), and that of the DNA synthetic phase (Ts=9.4 h) is derived from the y-interceptTs/Tc=0.3301.Tc–Ts is the time needed to reach the maximum labelling value. The length of the G2/M phase was calculated using the following equation: TG2/M=(% Histone H3–P+CBC cells×Tc). Figure 2: Cytokinetic parameters of CBC cells. ( a ) Schematic representation of the protocol of cumulative CldU labelling. The solid black line represents the length of the S phase relative to the other phases of the cycle. The solid red line represents the distribution of cells within the cycle, which have been labelled with CldU. ( b ) Kinetics of cumulative CldU incorporation in CBC stem cells. We performed CldU immunohistochemistry on thin paraffin sections of rolled intestine, using Ki67 as a marker of cycling cells and phospho (ser10)-histone H3 to evaluate the percentage of cells in the G2/M transition. Analysis of the relationship between the ratio of CldU + Ki67 + CBC cells to the total number of Ki67 + CBC cells and time revealed a linear increase in labelled CBC cells until CldU labelling became saturated. Data points represent mean percentages of Ki67 + CldU + CBC cell nuclei from two mice (A-F and I-M), except for the 21-h and 25-h time points (mice G,H). The average length of the cell cycle ( T c=28.5 h) is given by the slope of the regression line (1/0.0351), and that of the DNA synthetic phase ( T s=9.4 h) is derived from the y-intercept T s/ T c=0.3301. T c– T s is the time needed to reach the maximum labelling value. The length of the G2/M phase was calculated using the following equation: TG2/M=(% Histone H3–P + CBC cells× T c). Full size image CBC and cp4 cells segregate chromosomes randomly In addition to the cell cycle length and the CS mode (random versus nonrandom), the rate of decrease in the proportion of labelled cell nuclei should also depend on the rate of migration of the cell progeny out of the stem compartment, and the threshold of label detection δ . We built a mathematical model that integrates all the parameters cited above, the predictions of which are shown in Fig. 3a–d (see Methods). According to this model, nonrandom CS should easily be distinguished from random CS by examining the time-dependent decrease in the proportion of CldU + CBC cells, starting from a fully labelled cell population, and provided that δ is equal or inferior to 0.25 labelled strand per chromosome (see Methods). This threshold allows the detection of cells in which at least one-fourth of the chromosomes contain one labelled strand (green curves in Fig. 3c,d ). Indeed, if these conditions are met, very few labelled nuclei should be detected in crypt bottoms after three days of chase (>2 generations) in case of nonrandom CS ( Fig. 3c ), whereas over 90% labelled CBC cell nuclei should still be detected in the case of random CS ( Fig. 3d ). 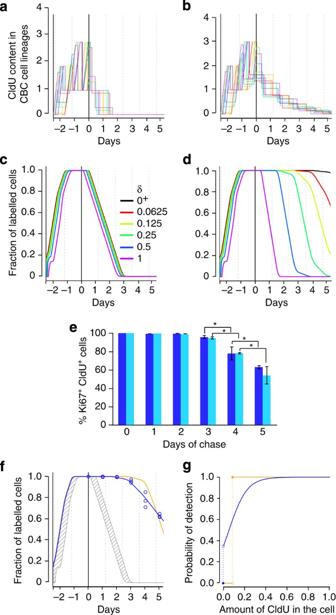Figure 3: Analysis of the CBC and cp4 cell-modes of chromosome segregation during a labelling-dilution experiment. (a,b) Simulation of the CldU content fluctuations in ten individual CBC cell lineages (one colour per lineage) during a pulse-chase experiment. A CldU content beyond 2 cannot be reached before the beginning of the S phase, when ploidy increases. (a) In the case of nonrandom CS, the number of labelled DNA strands per chromosome (CldU content) should substantially increase after 2 days of labelling (−2 to 0) but should decrease abruptly within 2–3 days of chase. (b) In the case of random CS, the CldU content should decay at a slower rate and labelled DNA should still be present after 5 days of chase. (c,d) Mathematical modelling of the DNA label dilution kinetics. The proportion of CldU+cells depends on the minimal amount of CldU-labelled DNA that can be detected by immunofluorescence. The parameterδcorresponds to this threshold in our simple detection model25. Predictions are represented for the nonrandom and random CS scenarios and six thresholds of detection ranging fromδ=1 (CldU content >one labelled strand per chromosome) to the limit whenδapproaches 0 (black line perfect detection). (c) In the case of nonrandom CS, CldU should be lost from the stem cell compartment after 3 days of chase, whereas in the case of random CS (d), CldU should still be present and detected provided thatδ<0.5. (e) Kinetics of CldU dilution in the fully labelled CBC (dark blue) and cp4 (turquoise blue) cell populations. Mean±s.d. (n=3). One initial injection of CldU was followed by CldU in drinking water for 60 h (>2Tc). Mice were killed at the end of the labelling period and every day for 5 consecutive days. The differences between day 4 and day 3 and between day 5 and day 4 are significant (P< 0.05, Fisher's exact test). (f) Model fit for CBC cells. The observed kinetics (data represented by open circles) is compared with the nonrandom CS scenario (grey hatched area) and the random CS scenario after estimating the label-detection threshold (orange line) and a more sophisticated two-parameter model of label detection (blue line). The fraction of variance (r2) explained by this second model reaches 0.96 compared with 0.74 with the simple model. (g) Modelling the probability of label detection as a function of the CldU content. The orange line represents the probability of detection, using the simple model estimated on the experimental data (δ=0.088). The second model represented by the blue line accounts for randomness in the detection process. It involves two parameters,δandɛ, estimated from the experimental data (δ=0.055 andɛ=0.085). Figure 3: Analysis of the CBC and cp4 cell-modes of chromosome segregation during a labelling-dilution experiment. ( a , b ) Simulation of the CldU content fluctuations in ten individual CBC cell lineages (one colour per lineage) during a pulse-chase experiment. A CldU content beyond 2 cannot be reached before the beginning of the S phase, when ploidy increases. ( a ) In the case of nonrandom CS, the number of labelled DNA strands per chromosome (CldU content) should substantially increase after 2 days of labelling (−2 to 0) but should decrease abruptly within 2–3 days of chase. ( b ) In the case of random CS, the CldU content should decay at a slower rate and labelled DNA should still be present after 5 days of chase. ( c , d ) Mathematical modelling of the DNA label dilution kinetics. The proportion of CldU + cells depends on the minimal amount of CldU-labelled DNA that can be detected by immunofluorescence. The parameter δ corresponds to this threshold in our simple detection model [25] . Predictions are represented for the nonrandom and random CS scenarios and six thresholds of detection ranging from δ =1 (CldU content >one labelled strand per chromosome) to the limit when δ approaches 0 (black line perfect detection). ( c ) In the case of nonrandom CS, CldU should be lost from the stem cell compartment after 3 days of chase, whereas in the case of random CS ( d ), CldU should still be present and detected provided that δ <0.5. ( e ) Kinetics of CldU dilution in the fully labelled CBC (dark blue) and cp4 (turquoise blue) cell populations. Mean±s.d. ( n =3). One initial injection of CldU was followed by CldU in drinking water for 60 h (>2Tc). Mice were killed at the end of the labelling period and every day for 5 consecutive days. The differences between day 4 and day 3 and between day 5 and day 4 are significant ( P < 0.05, Fisher's exact test). ( f ) Model fit for CBC cells. The observed kinetics (data represented by open circles) is compared with the nonrandom CS scenario (grey hatched area) and the random CS scenario after estimating the label-detection threshold (orange line) and a more sophisticated two-parameter model of label detection (blue line). The fraction of variance ( r 2 ) explained by this second model reaches 0.96 compared with 0.74 with the simple model. ( g ) Modelling the probability of label detection as a function of the CldU content. The orange line represents the probability of detection, using the simple model estimated on the experimental data ( δ =0.088). The second model represented by the blue line accounts for randomness in the detection process. It involves two parameters, δ and ɛ , estimated from the experimental data ( δ =0.055 and ɛ =0.085). Full size image Using the timeframe predicted by our model, we designed a DNA labelling–dilution experiment. To avoid the stress inflicted by repeated injections, adult mice were administered one initial injection of CldU, followed by CldU in drinking water for 2.5 days ( ∼ 2 generations), a duration that we knew was more than sufficient to label 100% cells. Using CldU instead of BrdU allowed us to pulse mice with IdU at the end of the labelling period, and we found that the proportion of CBC cells transiting through the DNA S phase (36%) was unchanged compared with untreated control mice. For cell scoring, we distinguished Ki67 + CBC cells flanked by Paneth cells from the first Ki67 + located above the last Paneth cells, at the average +4 position (cp4) from the base [24] . The results show that after 2 days of chase, which exceeds the time required to complete the first round of cell divisions in the absence of label, a CldU signal is detected in nearly 100% of CBC and cp4 cells ( Fig. 3e and Supplementary Table S1 ). By day 3, all cells have been through two successive divisions in the absence of label and yet a clear signal can be detected in 94–97% of CBC cells and 93–96% of cp4 cells ( Fig. 3e ). These experimental data are incompatible with the nonrandom CS segregation scenario and are instead in broad agreement with the predictions of the random CS model, with a detection threshold of 0.09 labelled strand per chromosome ( Fig. 3f , orange line, r 2 =0.74). The observed kinetics of label dilution nevertheless suggests that modelling the detection of the label using a single parameter ( δ ) [25] is oversimplified (orange line in Fig. 3g ). Realistically, other factors than the amount of label in the cell should influence the results, such as the orientation of the cell relative to the crypt section. Therefore, the data are better explained with a two-parameter model accounting for some degree of randomness in the decision of calling a cell CldU + ( Fig. 3f,g , blue lines, r 2 =0.96). As illustrated in Fig. 4 , the CldU-labelling pattern changed from bright and homogeneous at the end of the labelling period (T0) to spotty after 24 h in the absence of CldU. The largest CldU-labelled spots ( Fig. 4i–k ) likely correspond to clusters of major and minor satellite repeats of centromeres (also called chromocenters) that remain associated through interphase and S phase, and dissociate only in prophase [26] , [27] . Between 1 and 3 days of chase ( Fig. 4h–j ), the number but not the intensity of the spots steadily decreased, attesting the progressive loss of labelled chromosomes through successive divisions. Taken together, the results indicated that in the unlesioned epithelium of adult mice, CBC stem cells as well as cp4 cells segregate most if not all their chromosomes randomly. 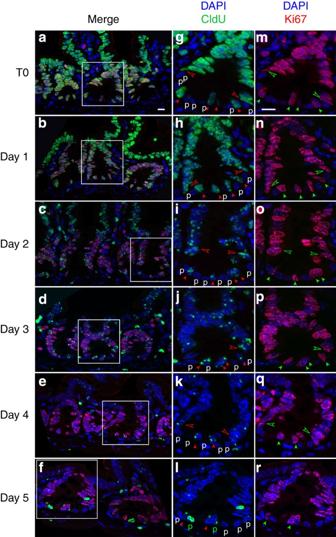Figure 4: CldU and Ki67 immunostaining of the CBC and cp4 cell populations. Mice were killed at the beginning of the chase period (T0) and every day for 5 consecutive days. (a–f) Merged lower power views of ileal crypt sections stained for CldU (green) and Ki67 (red), and counterstained with 4′-6-diamidino-2-phenylindole (DAPI) on (a) day 0, (b) day 1, (c) day 2, (d) day 3, (e) day 4 and (f) day 5. (g–r) Enlarged single-channel views of the crypt sections present in the insets. (g–l) CldU staining on (g) day 0, (h) day 1, (i) day 2, (j) day 3, (k) day 4 and (l) day 5. Note that the number but not the intensity of the spots steadily decreased from T0 (g) to day 5 (l), attesting the progressive loss of labelled chromosomes through successive divisions. (m–r) Ki67 staining on (m) day 0, (n) day 1, (o) day 2, (p) day 3, (q) day 4 and (r) day 5. Closed and open arrowheads point to CBC cell and cp4 cell nuclei, respectively. P, unlabelled (white) and CldU-labelled (green) Paneth cell nuclei. Scale bars, 10 μm. Figure 4: CldU and Ki67 immunostaining of the CBC and cp4 cell populations. Mice were killed at the beginning of the chase period (T0) and every day for 5 consecutive days. ( a – f ) Merged lower power views of ileal crypt sections stained for CldU (green) and Ki67 (red), and counterstained with 4′-6-diamidino-2-phenylindole (DAPI) on ( a ) day 0, ( b ) day 1, ( c ) day 2, ( d ) day 3, ( e ) day 4 and ( f ) day 5. ( g – r ) Enlarged single-channel views of the crypt sections present in the insets. ( g – l ) CldU staining on ( g ) day 0, ( h ) day 1, ( i ) day 2, ( j ) day 3, ( k ) day 4 and ( l ) day 5. Note that the number but not the intensity of the spots steadily decreased from T0 ( g ) to day 5 ( l ), attesting the progressive loss of labelled chromosomes through successive divisions. ( m – r ) Ki67 staining on ( m ) day 0, ( n ) day 1, ( o ) day 2, ( p ) day 3, ( q ) day 4 and ( r ) day 5. Closed and open arrowheads point to CBC cell and cp4 cell nuclei, respectively. P, unlabelled (white) and CldU-labelled (green) Paneth cell nuclei. Scale bars, 10 μm. Full size image CBC and cp4 cells are not LRCs There are several reports on the capacity of stem cells of the adult small intestinal epithelium to retain DNA label for long periods of time during the period of regeneration that follows a lesion [4] , [28] , [29] , [30] . Although a clear correlation between cell position and differentiation or proliferation of LRCs was not evident in these studies, long-term label retention has been considered until now as the exclusive property of stem cells in the epithelium of the small intestine [4] , [28] , [29] , [30] . We therefore decided to perform a label retention assay that includes an IHC technique (see Methods) capable of discriminating putative cycling or quiescent undifferentiated LRCs from post-mitotic differentiated LRCs present in the crypt base (Paneth, entero-endocrine and tuft cells [12] ). To be as discriminatory as possible in the detection of stem cells, we used Lgr5-EGFP mice [15] in which GFP is expressed in 20–30% of the crypts and cycling CBC cells sandwiched between Paneth cells are GFP high [15] . Lgr5-EGFP mice were irradiated with a dose of 6 Gy of Cs 137 to the whole body, after which mice were administered BrdU in drinking water for 5 days. Control and irradiated mice were killed 2, 5, 14 and 23 days post irradiation. Both GFP + and GFP − CBC cells were counted and the data pertaining to this experiment can be found in Supplementary Tables S2-S5 . The efficiency of irradiation was attested at day 2 by a significant decrease in the number of GFP + crypt sections ( Fig. 5a ) and in the number of Ki67 + CBC cells ( Fig. 5b ), whereas the Ki67 + cp4 cell score was unchanged ( Fig. 5b ). The complete recovery of GFP expression and CBC cells was observed 5 days post irradiation ( Fig. 5a,b ). In addition, the CBC and cp4 cell populations were fully labelled as in control mice ( Fig. 5c ). Fluorescent photomicrographs acquired at low as well as high magnification illustrate the radiation-induced changes in the CBC cell population observed during the BrdU-labelling period ( Fig. 6 ). As predicted by the model of random CS ( Supplementary Fig. S1 ), BrdU + CBC and BrdU + cp4 cells could still be detected after 9 days of chase but not at day 23 after 18 days of chase ( Fig. 7 ). After 9 days of chase (day 14 post-irradiation), two types of BrdU + nuclei were present in the stem compartment and could easily be distinguished on the basis of the intensity and staining pattern. Both in GFP + and GFP − crypts, all BrdU high nuclei without exception belonged to post-mitotic lineage + cells, whereas BrdU low nuclei were predominantly found in CBC or cp4 cells at a frequency expected in case of random CS after eight cell generations ( Fig. 7 ). In line with their relatively longer turnover time (8 weeks) [31] , Paneth cell nuclei were over-represented in the BrdU high group, compared with entero-endocrine and tuft cells, with turnover times of 4–10 days [32] , [33] ( Fig. 7 and Supplementary Table S5 ). 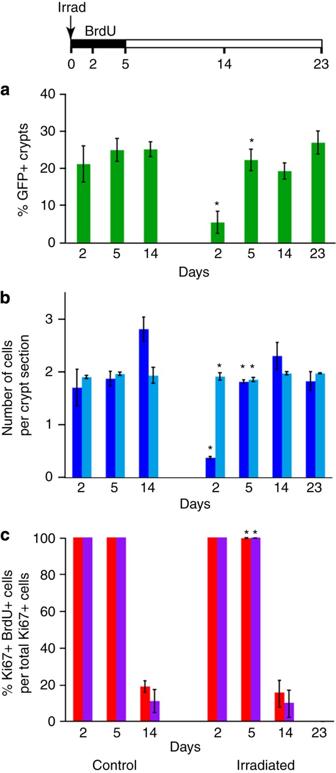Figure 5: Quantification of CBC cell depletion, followed by recovery in the ileum of irradiated mice. Lgr5-EGFP mice were irradiated (or not) with a dose of 6 Gy of Cs137to the whole body. They were then administered BrdU in drinking water for 5 days and killed 2, 5, 14 and 23 days post irradiation. (a) Temporary decrease followed by recovery in GFP expression in the crypt epithelium of irradiated mice. (b) Transient irradiation-induced depletion in CBC cells (dark blue) but not cp4 cells (turquoise blue) 2 days post irradiation. (c) Similar rates of BrdU incorporation (day 5) and BrdU dilution (day 14) in CBC cells (red) and cp4 cells (purple) in irradiated versus control mice. Note that 2 days post irradiation, 100% of surviving CBC cells were Ki67+BrdU+. Data are presented as mean with error bars. Error bars with * (n=3) correspond to standard deviations and bars without * (n=2) indicate the range. The values obtained from distinct mice for the same time point (seeSupplementary Tables S2-S5) were compared using Fisher's exact test. Figure 5: Quantification of CBC cell depletion, followed by recovery in the ileum of irradiated mice. Lgr5-EGFP mice were irradiated (or not) with a dose of 6 Gy of Cs 137 to the whole body. They were then administered BrdU in drinking water for 5 days and killed 2, 5, 14 and 23 days post irradiation. ( a ) Temporary decrease followed by recovery in GFP expression in the crypt epithelium of irradiated mice. ( b ) Transient irradiation-induced depletion in CBC cells (dark blue) but not cp4 cells (turquoise blue) 2 days post irradiation. ( c ) Similar rates of BrdU incorporation (day 5) and BrdU dilution (day 14) in CBC cells (red) and cp4 cells (purple) in irradiated versus control mice. Note that 2 days post irradiation, 100% of surviving CBC cells were Ki67 + BrdU + . Data are presented as mean with error bars. Error bars with * ( n =3) correspond to standard deviations and bars without * ( n =2) indicate the range. The values obtained from distinct mice for the same time point (see Supplementary Tables S2-S5 ) were compared using Fisher's exact test. 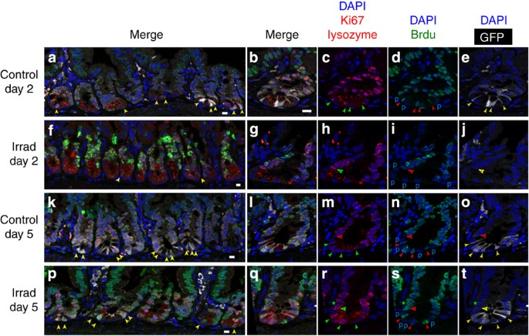Figure 6: Immunofluorescence CBC cell BrdU-labelling at 2 and 5 days post irradiation. Control (a–e,k–o) and irradiated (f–j,p–t) Lgr5-EGFP mice were continuously exposed to BrdU administered in drinking water and killed after 2 and 5 days. Ileum sections were simultaneously stained for nuclear BrdU (green), nuclear Ki67 (red), cytoplasmic lysozyme (red) and cytoplasmic green fluorescent protein (GFP, white). Nuclei were counterstained with DAPI (blue). Closed and open arrowheads point at CBC and to cp4 cells, respectively. (a) Merge picture of neighbouring GFP+and GFP−crypt sections. (b) Merge picture of a crypt section with four CBC cells staining positive for Ki67 (c, green arrowheads) BrdU (d, red arrowheads) and GFP (e, yellow arrowheads). (f) Merge picture of crypt sections devoid of CBC cells. (g) Merge picture of a single crypt section. The cp4 cell of this crypt (open arrowhead) is Ki67+(h), BrdU+(i) and GFP−(j). (k) Merge picture of GFP+crypt sections. (l) Merge picture of a single crypt section with four CBC cells and one cp4 cell, all of which are Ki67+(m), BrdU+(n) and GFP+(o). (p) Merge picture of a succession of GFP+and GFP−crypt sections. (q) Merge picture of a single GFP+crypt section with four CBC cells, all of which are Ki67+(r), BrdU+(s) and GFP+(t). Note the presence of a Ki67+BrdU+GFP−cp4 cell and the BrdU+Ki67−nucleus (*) of a post-mitotic cell sandwiched between Ki67+BrdU+progenitor nuclei. P, Paneth cell nuclei. Scale bar, 10 μm. DAPI, 4′-6-diamidino-2-phenylindole. Full size image Figure 6: Immunofluorescence CBC cell BrdU-labelling at 2 and 5 days post irradiation. Control ( a–e , k – o ) and irradiated ( f – j , p – t ) Lgr5-EGFP mice were continuously exposed to BrdU administered in drinking water and killed after 2 and 5 days. Ileum sections were simultaneously stained for nuclear BrdU (green), nuclear Ki67 (red), cytoplasmic lysozyme (red) and cytoplasmic green fluorescent protein (GFP, white). Nuclei were counterstained with DAPI (blue). Closed and open arrowheads point at CBC and to cp4 cells, respectively. ( a ) Merge picture of neighbouring GFP + and GFP − crypt sections. ( b ) Merge picture of a crypt section with four CBC cells staining positive for Ki67 ( c , green arrowheads) BrdU ( d , red arrowheads) and GFP ( e , yellow arrowheads). ( f ) Merge picture of crypt sections devoid of CBC cells. ( g ) Merge picture of a single crypt section. The cp4 cell of this crypt (open arrowhead) is Ki67 + ( h ), BrdU + ( i ) and GFP − ( j ). ( k ) Merge picture of GFP + crypt sections. ( l ) Merge picture of a single crypt section with four CBC cells and one cp4 cell, all of which are Ki67 + ( m ), BrdU + ( n ) and GFP + ( o ). ( p ) Merge picture of a succession of GFP + and GFP − crypt sections. ( q ) Merge picture of a single GFP + crypt section with four CBC cells, all of which are Ki67 + ( r ), BrdU + ( s ) and GFP + ( t ). Note the presence of a Ki67 + BrdU + GFP − cp4 cell and the BrdU + Ki67 − nucleus (*) of a post-mitotic cell sandwiched between Ki67 + BrdU + progenitor nuclei. P, Paneth cell nuclei. Scale bar, 10 μm. DAPI, 4′-6-diamidino-2-phenylindole. 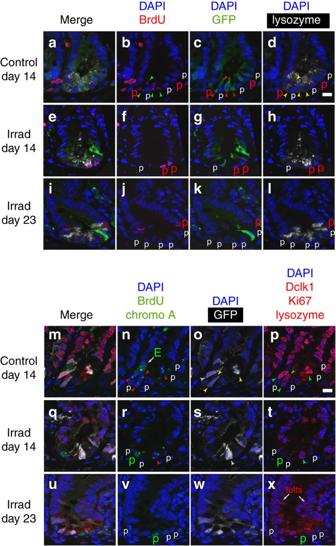Figure 7: CBC and cp4 cells of irradiated Lgr5-EGFP mice are not label-retaining cells. Control and irradiated Lgr5-EGFP mice were continuously exposed to BrdU for 5 days and killed 14 days (9 days of chase) and 23 days (18 days of chase) after the beginning of the treatment. Ileum sections were either simultaneously stained for BrdU, GFP and lysozyme (a–l) or BrdU, GFP, lysozyme, chromogranin A, Dclk1 and Ki67 (m–x). (a–d) Single crypt section from a control mouse. (a) Merge. (b) BrdU+CBC cell nuclei (green arrowheads) sandwiched between BrdU+and BrdU−Paneth cell nuclei (p). The CBC cells of this crypt section are all GFP+(arrowheads inc) and the Paneth cells are lysozyme+(d). (e–h) Single crypt section from an irradiated mouse killed 14 days post irradiation. (e) Merge. The two nuclei that stain positive for BrdU (f) and negative for GFP (g) belong to Paneth cells with cytoplasmic lysozyme granules (h). (i–l) Single crypt section from an irradiated mouse killed 23 days post irradiation. (i) Merge. The BrdU+nucleus (j) belongs to a GFP−(k) lysozyme+(l) Paneth cell. (m–p) Single crypt from a control mouse. (m) Merge. (n) The small arrow points at an entero-endocrine cell (E) with nuclear BrdU and cytoplasmic chromogranin A staining. Arrowheads point at BrdU+nuclei that belong to GFP+(o), KI67+(p) CBC cells. (q–t) Single crypt section from an irradiated mouse killed 14 days post irradiation. (q) Merge. (r) Two BrdU+nuclei, one of which belongs to a GFP+cell (arrowhead ins) and the other to a lysozyme+Paneth cell (t). (u–x) Single crypt section from an irradiated mouse killed 23 days post irradiation. (u) Merge. (v) The BrdU+nucleus belongs to a GFP−(w) lysozyme+(x) Paneth cell. White arrows in (x) point at BrdU−Dclk1+tuft cells. Scale bar, 10 μm. DAPI, 4′-6-diamidino-2-phenylindole. Full size image Figure 7: CBC and cp4 cells of irradiated Lgr5-EGFP mice are not label-retaining cells. Control and irradiated Lgr5-EGFP mice were continuously exposed to BrdU for 5 days and killed 14 days (9 days of chase) and 23 days (18 days of chase) after the beginning of the treatment. Ileum sections were either simultaneously stained for BrdU, GFP and lysozyme ( a – l ) or BrdU, GFP, lysozyme, chromogranin A, Dclk1 and Ki67 ( m – x ). ( a – d ) Single crypt section from a control mouse. ( a ) Merge. ( b ) BrdU + CBC cell nuclei (green arrowheads) sandwiched between BrdU + and BrdU − Paneth cell nuclei (p). The CBC cells of this crypt section are all GFP + (arrowheads in c ) and the Paneth cells are lysozyme + ( d ). ( e – h ) Single crypt section from an irradiated mouse killed 14 days post irradiation. ( e ) Merge. The two nuclei that stain positive for BrdU ( f ) and negative for GFP ( g ) belong to Paneth cells with cytoplasmic lysozyme granules ( h ). ( i – l ) Single crypt section from an irradiated mouse killed 23 days post irradiation. ( i ) Merge. The BrdU + nucleus ( j ) belongs to a GFP − ( k ) lysozyme + ( l ) Paneth cell. ( m – p ) Single crypt from a control mouse. ( m ) Merge. ( n ) The small arrow points at an entero-endocrine cell (E) with nuclear BrdU and cytoplasmic chromogranin A staining. Arrowheads point at BrdU + nuclei that belong to GFP + ( o ), KI67 + ( p ) CBC cells. ( q – t ) Single crypt section from an irradiated mouse killed 14 days post irradiation. ( q ) Merge. ( r ) Two BrdU + nuclei, one of which belongs to a GFP + cell (arrowhead in s ) and the other to a lysozyme + Paneth cell ( t ). ( u – x ) Single crypt section from an irradiated mouse killed 23 days post irradiation. ( u ) Merge. ( v ) The BrdU + nucleus belongs to a GFP − ( w ) lysozyme + ( x ) Paneth cell. White arrows in ( x ) point at BrdU − Dclk1 + tuft cells. Scale bar, 10 μm. DAPI, 4′-6-diamidino-2-phenylindole. Full size image Before Lgr5 was coined as a specific marker of intestinal epithelial stem cells [15] , CBC cells were known to be more radiosensitive, to cycle more slowly and not to display the circadian rhythm evident for cells at higher positions, suggesting that they represent a distinct cell population (reviewed in refs 12 , 34 ). Here we confirmed that, at least in the small intestine, CBC cells do represent a single population in terms of proliferation kinetics and in terms of radiosensitivity. The return to a normal number of CBC cells within 5 days post irradiation highlights the outstanding capacity of the crypt to respond to acute damage by recruiting surviving CBC cells or progenitors of the transit-amplifying zone so as to replenish the stem-cell pool. The results of our label dilution and label retention assays suggest that intestinal epithelial stem cells segregate most if not all their chromosomes randomly, both under homeostatic conditions and when recovering from a lesion. In addition, we demonstrate that unlike what is commonly thought, all label-retaining cells found in the lower half of the crypts 18 days after irradiation are post-mitotic, terminally differentiated cells, and that cycling cp4 cells are not LRCs. The observed longer retention of BrdU in Paneth cell nuclei compared with CBC cells and other types of differentiated cells was expected considering the slow rate of Paneth cell replacement compared with the other cell types. With the type of pulse-chase experiments used to test the immortal strand hypothesis in our study and in previous studies, it is difficult to answer the question of whether one or a small number of chromosomes segregate asymmetrically, a potential mechanism proposed by others to regulate lineage cell commitment [3] , [8] . This question was recently addressed in the unlesioned mouse colon epithelium, using the technique of chromosome orientation fluorescent in situ hybridization to follow the fate of parental template strand inheritance in mitotic cell pairs [35] . Because the orientation of major satellite DNA relative to telomeric DNA is fixed, probes hybridized to major satellite repeats were used to arbitrarily define a Watson (major A-rich satellite) and a Crick (major T-rich satellite) DNA template. The results revealed a higher frequency of daughter-cell pairs with asymmetry, than predicted by simulated random segregation. This was interpreted as a possible indication that nonrandom CS contributes to cell-fate decisions [35] . However, CS could, in theory, be nonrandom with respect to chromosome orientation (that is, all Crick or all Watson strands inherited by the same daughter cell) and yet, cell fate be independent of this phenomenon. Conversely, if retention of the same parental template strand of one or several chromosomes is linked to cell fate, and if this mechanism is independent of DNA orientation, the current chromosome orientation fluorescent in situ hybridization method could not possibly detect it. We have examined some possible scenarios that deviate from the purely random CS model and consider the possibility of nonrandom CS concerning a fraction of chromosomes, or occurring in a fraction of the cell population ( Supplementary Fig. S2 and Supplementary Discussion ). Whereas rare occurrences of either scenario cannot be completely ruled out, we reached the conclusion that to be compatible with our data and the sensitivity of our technique (detection in the transit amplifying zone after 3 days of chase, that is, after five rounds of division and a 32-fold dilution of the label), the fraction of cells or chromosomes subjected to nonrandom CS would have to be small in order to escape detection in the post-irradiation label retention assay. Our post-irradiation label retention assay is the first of the kind in which a clear correlation between cell position, differentiation and proliferation for each label-retaining and each non-LRC could be established among the hundreds of cells examined. A significant point of concern regarding previous studies was the lack of reference to Ki67 or PCNA staining, which could have been used to unambiguously establish the proliferative status of LRCs [4] , [28] , [29] , [30] . In one instance, the close proximity of labelled and unlabelled nuclei was used to distinguish mitotic pairs from unrelated nuclei in wholemount preparations [30] . However, in our opinion, deciding whether two nuclei form a mitotic pair or belong to neighbouring cells are difficult distinctions to make in situ , when based only on the distance between nuclei. In contrast, the distance between nuclei is a valid parameter when looking at dividing cells in vitro [6] , [7] , [8] . We assume that the differences listed above between our experimental setup and that of previous studies could explain why we reached substantially different conclusions. Importantly, our results agree with the conclusion of two recent studies in which monoclonal conversion of intestinal epithelial crypts was analysed at single stem cell resolution [36] , [37] . In both studies, clone-size expansion or contraction was observed before monoclonal conversion was complete, and this early dynamics was found to have the 'scaling' behaviour expected for a scenario of neutral drift within a population of stem cells. According to their data the authors state that if the population size is 14–18, a figure they believe to be likely, then symmetric divisions in which both stem cell daughters have the same fate should be the rule rather than the exception [36] , [37] , and this argues against long-term template-strand retention in the stem-cell lineage. In conclusion, similar to what was previously demonstrated for the haematopoietic system and the skin [25] , [38] , [39] , both tissues undergoing continuous turnover during adult life and engaged in wound repair in response to injury, our study does not support the chromosome-sorting model as a major mechanism of genome integrity preservation in the adult intestinal epithelium. Mice and chemicals Adult (13- to 16-week old) male C57BL/6 mice were purchased from Charles River Laboratories (Arbresle, France) and housed under standard laboratory conditions on a light–dark cycle of 0800 to 2000 hours of light, with free access to food and water. Lgr5-EGFP-IRES-creERT2 (Lgr5-EGFP) mice were provided by Dr Eduard Batlle at the Institute for Research in Biomedicine of Barcelona, Spain. Experiments were performed according to the principles of laboratory animal care in compliance with the European and French law. Chemicals and antibodies are listed in Supplementary Methods and Supplementary Table S6 . Measurement of CBC cell cytokinetic parameters Adult C57BL/6 mice were administered five successive intraperitoneal injections of CldU (35 mg per kg of body weight) in Hanks buffered saline solution at 3- or 4-h intervals for a total period of 24 h. The first and last injections were administered at 0700 h. Two mice were killed 1 h after each CldU injection. The small intestine was flushed with phosphate-buffered saline (PBS) and 10-cm long segments were everted on 3-mm OD wooden skewers before fixation in 3% paraformaldehyde (PFA) for 3 h, followed by overnight incubation in ice-cold PBS. Intestines were released from the skewers by a longitudinal incision and rolled up using wooden toothpicks. Rolls were then processed for IHC on paraffin sections, according to standard protocols [40] . Thin (1–2 μm) sections were stained for CldU and Ki67, and the proportions of Ki67 + CldU + and CldU − CBC cell nuclei were determined from a collection of fluorescence images acquired with a Zeiss Axio Imager microscope equipped with a ×40 objective and an ApoTome slider. CldU-labelling-dilution and CldU-IdU double labelling assays Adult C57BL/6 mice were administered one initial intraperitoneal injection of 32.56 mM CldU in Hanks buffered saline solution (85.5 mg per kg of body weight), followed by CldU in drinking water (1 mg ml −1 ) for 60 h, a duration that is more than sufficient to label 100% CBC cells. The lack of cytotoxicity induced by continuous CldU exposure was attested, after one IP injection of 32.56 mM IdU (115.3 mg kg −1 of body weight), by the unchanged level of nuclear cleaved caspase 3, compared with untreated control mice (not shown) and the unchanged proportion (36%) of CBC cells transiting through the DNA S phase. This procedure was adapted from a previously described protocol [41] . Antigen retrieval in 10 mM sodium citrate buffer, pH 6.0 for 20 min, was not followed by incubation with HCl (2 N). Incubation with the primary antibodies overnight at 4 °C was followed by incubation with 0.5 M NaCl for 6 min to eliminate nonspecific binding of the anti-IdU antibody. The anti-Ki67 and anti-lysozyme antibodies were then reapplied for 1 h at room temperature before rinsing in PBS-Tween and incubation for 1 h at room temperature with secondary antibodies [41] . BrdU-labelling during post-irradiation crypt regeneration Lgr5-EGFP mice were administered one initial injection of BrdU (60 mg kg −1 ) followed (or not) by irradiation with a dose of 6 Gy of Cs 137 to the whole body (3.5 Gy min −1 ), with a therapeuthic irradiator. They were then administered BrdU in drinking water (1 mg ml −1 ) for 5 days and groups of control and irradiated mice were killed 2, 5, 14 and 23 days post irradiation. CBC and cp4 cell scoring procedure For cell scoring, we distinguished Ki67 + CBC cells flanked by Paneth cells from the first Ki67 + located above the last Paneth cells, at the average +4 position (cp4) from the base [24] . To facilitate CBC cell spotting, we restricted our analysis to the ileum, at which the most abundant Paneth cell and CBC cell populations are found. As all CBC cell nuclei stain positive for Ki67, to determine the fraction of CBC cells with labelled nuclei (BrdU, CldU or IdU), the following criteria were applied during counting: CBC cell nuclei located between Paneth cells (not above) were scored; Ki67 + /BrdU + and Ki67 + /BrdU − nuclei were scored in well-oriented crypt sections, defined as crypts that contain a single layer of epithelial cells surrounding their lumen, and those that are adjacent to the muscularis mucosa. Two independent persons performed scoring. Scoring procedure for long-term BrdU-retaining cell nuclei We performed IHC on thin paraffin sections of rolled intestine, using antibodies directed against GFP and Ki67 (cycling cells), BrdU, and a cocktail of primary antibodies directed against lineage-specific antigens: chromogranin A for entero-endocrine cells; doublecortin-like kinase 1 (Dclk1) for tuft cells [11] ; and lysozyme for Paneth cells. A donkey anti-sheep-A488 conjugate was used to detect nuclear BrdU and cytoplasmic chromogranin A in entero-endocrine cells. A donkey anti-rabbit-Cy3 conjugate was used to detect nuclear Ki67, lysozyme + granules in the cytoplasm of Paneth cells and cytoplasmic dclk1 in tuft cells. Revealing several antigens with a single conjugate was possible because of the different subcellular localizations of the antigens (nuclear/cytoplasmic, diffuse cytoplasmic/cytoplasmic granules), and because each labelled cell could be unambiguously identified by its shape and localization along the crypt–villus axis. Importantly, this procedure was absolutely required to minimize the risk of overlooking the presence of rare cycling or quiescent lineage-negative BrdU + cells. Statistical analysis Proportions of Ki67 + CBC and cp4 cells labelled with CldU or BrdU obtained from distinct mice for the same timepoint were compared using Fisher's exact test. When not statistically significantly different ( P -values>0.05), counts from distinct mice were aggregated before timepoint comparison, also based on Fisher's exact test. Stochastic modelling of the proportion of labelled CBC cells In the CldU label dilution assay, the expected proportions of CldU + CBC daughter cells under the random and nonrandom CS scenarios were estimated using Monte-Carlo simulations of stem cell lineages, according to the model we describe below. Additional information is provided in the Supplementary Methods and Supplementary Software . The length of the cell cycle has mean μ =28.5 h and standard deviation σ =2 h. The cell cycle is subdivided into three parts with respect to ploidy. The S phase (ploidy increases from 2 to 4) accounts for a fraction β S =9.4 h/28.5 h of the cycle. The time after the S phase (ploidy=4) accounts for β 2 =3.4 h/28.5 h of the cycle. The time before the S phase (ploidy=2) accounts for β 1 =1− β S − β 2 of the cycle. As the number of CBC cells per crypt does not vary significantly during the day, production of new cells is continuously compensated by upward migration of older cells during this time. The daughter cells cannot be distinguished from one another until one of them migrates, and both have thus been included in the final count. Given that the maximum amount of time spent by each new generation should not exceed the duration of the CBC cell cycle, we modelled the two daughter cells as remaining for the same length of time in the crypt base, which is the most unfavourable situation to distinguish random from nonrandom CS in our pulse-chase experiment. Just before the g th generation, the stem cell contains K =2 n +2 chromosomes ( n =19) made of two DNA strands: one strand was the template, whereas the other was synthesized during generation g −1. After completion of the S phase, the cell contains two copies of the K chromosomes but only one copy of each chromosome contains the template DNA strand of generation g −1. At the beginning of generation g +1, each daughter cell inherits one copy of the K chromosomes. For each chromosome, the copy that contains the template DNA strand of generation g −1 remains in the simulated stem cell lineage with a probability P . The random and nonrandom CS scenarios compared in this study correspond to P =0.5 and P =1, respectively ( Fig. 1a,d ). The amount of CldU incorporated into the cell DNA increases at a constant rate during the S phase and as our unit of measure, we used the average number of labelled strands per chromosome. Therefore, one unit corresponds to one labelled DNA strand per chromosome in a diploid cell (40 labelled strands in the mouse) and two units to either one labelled DNA strand per chromosome in a tetraploid cell (at the end of the S phase) or two labelled strands per chromosome in a diploid cell (80 labelled strands in both cases). Figure 3a,b illustrate the variations of CldU content in stem cell lineages simulated with this model. The parameter δ is the amount of labelled DNA that a cell must contain to be detected and scored as CldU + [25] . It is expressed in the unit of measure described above. The output of our simulations is the proportion of CldU + cells detected for δ varying between 0.0625 and 1. We used the simulations to estimate δ and to investigate the fit of a more realistic model that incorporates a certain level of randomness in the detection of the label by means of a second parameter ɛ ( Fig. 3f,g ). Modelling the post-irradiation BrdU dilution assay Computations were carried out by the same procedure as that for the CldU dilution assay. As stem cells are supposed to adopt a random mode of CS during tissue regeneration before resuming nonrandom CS, the dynamics of label incorporation were not simulated. For simplicity, we assumed that all chromosomes were fully labelled after 5 days of pulse. How to cite this article: Escobar, M. et al . Intestinal epithelial stem cells do not protect their genome by asymmetric chromosome segregation. Nat. Commun. 2:258 doi: 10.1038/ncomms1260 (2011).